Enhanced sea-ice export from the Arctic during the Younger Dryas The Younger Dryas cold spell of the last deglaciation and related slowing of the Atlantic meridional overturning circulation have been linked to a large array of processes, notably an influx of fresh water into the North Atlantic related to partial drainage of glacial Lake Agassiz. Here we observe a major drainage event, in marine sediment cores raised from the Lomonosov Ridge, in the central Arctic Ocean marked by a pulse in detrital dolomitic-limestones. This points to an Arctic-Canadian sediment source area with about fivefold higher Younger Dryas ice-rafting deposition rate, in comparison with the Holocene. Our findings thus support the hypothesis of a glacial drainage event in the Canadian Arctic area, at the onset of the Younger Dryas, enhancing sea-ice production and drifting through the Arctic, then export through Fram Strait, towards Atlantic meridional overturning circulation sites of the northern North Atlantic. The Last Glacial Maximum (LGM) was followed by a deglaciation sequence punctuated by millennial-scale events, notably Heinrich Event 1 and the Younger Dryas (YD). It is now generally accepted that both involved a significant reduction in the Atlantic meridional overturning circulation (AMOC) attributed to enhanced meltwater inputs into the North Atlantic [1] , [2] . The YD, spanning ~12,800 to ~11,700 cal years BP [3] , [4] 3,4 corresponds to a period of cold conditions within the general climate warming that occurred during the transition from the LGM to the Holocene [5] , [6] . Of a large array of potential trigger mechanisms of the YD event that have been put forth [5] , [6] , [7] , [8] , the most widely supported scenario involves a major drainage pulse from glacial Lake Agassiz [7] , which surrounded the southwestern sector of the Laurentide Ice Sheet (LIS). A debate persists with respect to the drainage route, either eastward, through the Great Lakes–St Lawrence system or, northward, through the Mackenzie River delta [9] , [10] , [11] , [12] , [13] , [14] , [15] . However, high-resolution model experiments by Condron and Winsor [16] suggest that any meltwater pulse and/or re-routing from these eastern and southeastern continental outlets would be dispersed into the subtropical North Atlantic, with a subsequently limited influence on the AMOC sites. In addition, Murton et al . [17] provided evidence for drainage of Lake Agassiz, through the Mackenzie River delta, during the critical time interval. Optically stimulated luminescence measurements in aeolian sands interbedded with coarse fluvial material, assigned to drainage pulses, yielded ages compatible with a YD assignment. These findings strongly support the northward route scenario originally advanced by Tarasov and Peltier [11] and further discussed by Teller and Boyd [18] . Polyak et al . [19] also invoked this Arctic trigger scenario, based on a sedimentary record from the Chukchi margin. However, only one single 18 O depleted value supports the extension of their record into the YD interval, not to mention uncertainties about the age model, because of an open debate about the reservoir age correction for Arctic Ocean palaeowaters. Thus no clear 'marine' evidence for a major drainage event in the Canadian Arctic, at the onset of the YD, has yet been found. Here we present evidence for such a drainage event, based on detailed sedimentological and geochemical investigations on a multicore and a trigger-weight core (henceforth MC-18 and TC-18) taken from a Lomonosov Intrabasin, in the central Arctic, at a water depth of ~2,500 m ( Fig. 1 ). Our data demonstrate enhanced transport of sea ice from Canadian Arctic source, in the central Arctic, and its export through Fram Strait to the North Atlantic. 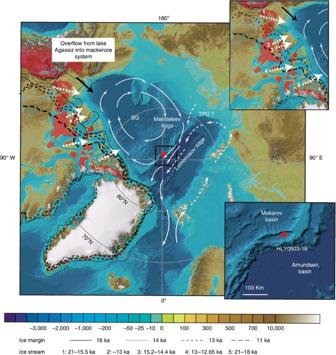Figure 1: Core location and geographical distribution of carbonates in Canadian Arctic region. The coring site HLY0503-18 is located on the Lomonosov Ridge in the central Arctic. Bathymetry is from the International Bathymetric Chart of the Arctic Ocean30. Mineralogical sources of calcite and dolomite (red areas) are indicated based on Phillips and Grantz24and the geological map of Canada. Palaeo-ice margins (black line) of the Laurentide Ice Sheet at 16, 14, 13 and 11 ka are represented with black line, and palaeo-ice streams are represented by white dashed arrows; approximate age are shown at the bottom of the figure, based on Dyke31and Stokes and Tarasov25. The Agassiz drainage route described by Murtonet al.17is indicated by the black arrow. Surface currents and sea-ice routes are represented by white arrows. We hypothesize an enhanced Beaufort Gyre (BG) during the Lake Agassiz drainage event through the Mackenzie area at ~13 to ~12 kaBP. Figure 1: Core location and geographical distribution of carbonates in Canadian Arctic region. The coring site HLY0503-18 is located on the Lomonosov Ridge in the central Arctic. Bathymetry is from the International Bathymetric Chart of the Arctic Ocean [30] . Mineralogical sources of calcite and dolomite (red areas) are indicated based on Phillips and Grantz [24] and the geological map of Canada. Palaeo-ice margins (black line) of the Laurentide Ice Sheet at 16, 14, 13 and 11 ka are represented with black line, and palaeo-ice streams are represented by white dashed arrows; approximate age are shown at the bottom of the figure, based on Dyke [31] and Stokes and Tarasov [25] . The Agassiz drainage route described by Murton et al . [17] is indicated by the black arrow. Surface currents and sea-ice routes are represented by white arrows. We hypothesize an enhanced Beaufort Gyre (BG) during the Lake Agassiz drainage event through the Mackenzie area at ~13 to ~12 ka BP . Full size image Chronology An age model based on eleven radiocarbon analyses on planktic foraminifer from TC-18, has been proposed by Hanslik et al . 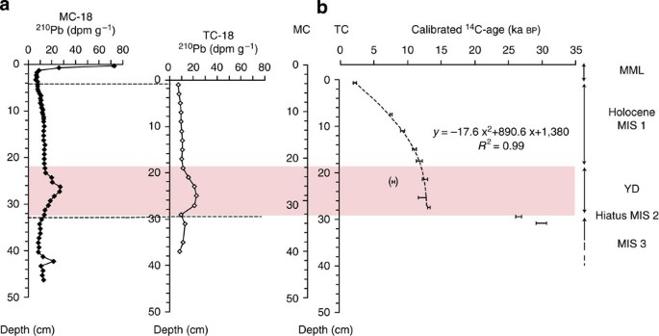Figure 2: Core age model. (a) Correlation between TC-18 and MC-18 based on210Pb data. (b) Chronology of MC-18 based on the age model of Hansliket al.20and210Pb correlation. The first three centimetres in MC-18 correspond to the modern mixed layer (MML; missing in TC-18). Down to 22 cm, the14C chronology suggests a sedimentation rate of 1.7 cm ka−1. The14C cluster from 22 to 33 cm (MC-18) with ages of ~13 to ~12 ka is assigned to the millennial-scale event of the YD age. Below 33 cm, the sequence indicates reduced sedimentation rates or even a hiatus during the LGM.14C-ages suggest a late MIS 3 assignment for sediments deposited before the YD event. The14C-outlier at 25 cm in MC-18 (bracketed), unexplained in Hansliket al.20, might be due to a non-local mixing event or a sampling artefact. Note the slight compaction with some smoothing of210Pb-activities in TC-18 compared with MC-18. The210Pb-peak assigned to the YD event matches a peak of parent230Th, whereas the top-1 cm peak in MC-18 relates mostly to the mixing of210Pb-rain produced in the water column during the last ~100 years. [20] High-resolution 210 Pb data allowed us to carry over this age model to MC-18 as illustrated in Figure 2 . The sedimentation rate is estimated to be 1.7 cm ka −1 during the Holocene. From ~22 to ~33 cm downcore, all ages fall into the range ~12 -13 cal ka BP , indicating a substantial increase in the rate of sedimentation during that period, combined with a 14 C-plateau [21] , which we attribute to the YD. Deeper in the core, two ages of almost 30 cal ka BP indicate a late Marine isotope stage (MIS) 3 assignment for the lower part of the section. The hiatus matching broadly the MIS 2 interval indicates either a near complete cessation of sediment supply, or its removal through erosion. Erosion seems improbable, because the coring site is located in a small intra-ridge basin. Thus, we interpret the abrupt jump from ~27 to ~13 cal ka BP (between ~34 and ~33 cm downcore in MC-18) as an indication of a near-complete cessation of sedimentation, thus of ice-rafting deposition, during MIS 2. This MIS 2-hiatus in sedimentation is also observed elsewhere in the central Arctic [22] and suggests reduced sea-ice mobility along the Beaufort Gyre and Transpolar Drift routes. Figure 2: Core age model. ( a ) Correlation between TC-18 and MC-18 based on 210 Pb data. ( b ) Chronology of MC-18 based on the age model of Hanslik et al . [20] and 210 Pb correlation. The first three centimetres in MC-18 correspond to the modern mixed layer (MML; missing in TC-18). Down to 22 cm, the 14 C chronology suggests a sedimentation rate of 1.7 cm ka −1 . The 14 C cluster from 22 to 33 cm (MC-18) with ages of ~13 to ~12 ka is assigned to the millennial-scale event of the YD age. Below 33 cm, the sequence indicates reduced sedimentation rates or even a hiatus during the LGM. 14 C-ages suggest a late MIS 3 assignment for sediments deposited before the YD event. The 14 C-outlier at 25 cm in MC-18 (bracketed), unexplained in Hanslik et al . [20] , might be due to a non-local mixing event or a sampling artefact. Note the slight compaction with some smoothing of 210 Pb-activities in TC-18 compared with MC-18. The 210 Pb-peak assigned to the YD event matches a peak of parent 230 Th, whereas the top-1 cm peak in MC-18 relates mostly to the mixing of 210 Pb-rain produced in the water column during the last ~100 years. Full size image Sedimentary and geochemical features A closer look at sedimentary and geochemical features allows the identification of the source and mechanism leading to the dispersal of detrital carbonates to the remote Lomonosov Ridge area during the subsequent YD interval. In the corresponding layer ( Fig. 3 ), carbonates are mainly composed of 50% calcite and 50% dolomite, which both increase in the silt and sand fractions ( Fig. 3 ). Such pulses of detrital, dolomite-rich carbonates are linked to the dispersal, off the LIS margin, of glacial sediments originating from Lower Palaeozoic bedrock areas, in the Canadian Arctic [23] , [24] . Palaeozoic carbonate rocks outcrop on Victoria Island, in the southern part of the Canadian Arctic Archipelago and in the Mackenzie Valley (based on the Canada Bedrock map, shown in Fig. 1 ). Three mechanisms can introduce detrital carbonates from these sources into the deep Arctic Ocean: erosion of carbonate glacial drift by melt water in the Mackenzie River drainage basin [17] ; density currents from LIS runoff along its northern margin; and ice-rafting from palaeo-ice streams (for example, from M'Clure Strait, carrying Silurian carbonate material from the NE Canadian margin [25] ). Enhanced ice-rafting from the eastern part of the Canadian Arctic Archipelago seems unlikely, as indicated by ice margin and ice stream palaeogeography at the onset of the YD ( Fig. 1 ). Moreover, a major peak in 230 Th-excess ( 230 Th xs ) matches this carbonate pulse, suggesting a strong influx of scavenging (thus relatively fine) particles ( Fig. 3 ). This excess, well above 230 Th-production by dissolved-U from the overlying water column, corresponds to a 230 Th xs flux about five times the mean Holocene flux ( Fig. 3 ). It indicates similarly enhanced fluxes of scavenging particles, in the sea-ice production areas, and supports the scenario of the long-distance ice-rafting dispersal of fine particles from the drainage event. Immediately above the corresponding sedimentary pulse, 230 Th xs decreases to its production in the overlying water column, thus indicating a drop in the sedimentary supply of scavenging particles. Later on, during the Holocene, 230 Th xs exceeding the overlying water column production is observed again, but with fluxes well below those highlighting the sedimentary pulse of the YD ( Fig. 3 ), a fact highlighting the singularity of the YD-event in the record. 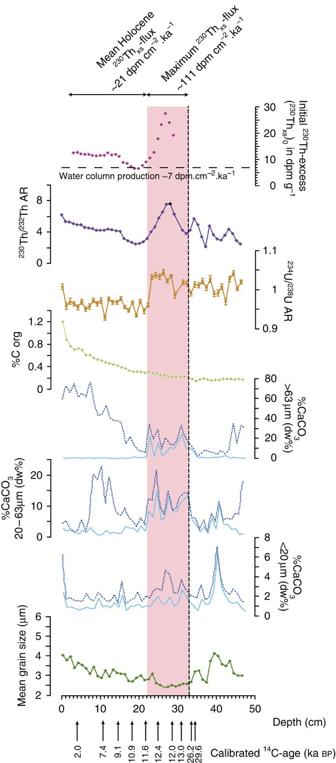Figure 3: Geochemical and sedimentological data for core HLY0503-18MC. 230Thxs0,230Th/232Th and234U/238U are respectively represented in pink, purple and orange. The mean grain size is represented in dark green, the organic carbon content in light green, dolomite and calcite are respectively in light and dark blue for all size fractions. The initial excess of230Th (230Thxs0) illustrated on top, represents the230Th produced through dissolved-234U decay in the water column and scavenged by sinking particles. It is calculated as the230Th in excess over the fraction supported by234U, in the sediment, with correction for radioactive decay since deposition. The horizontal dashed-line illustrating the230Th-production in the overlying water column is calculated on the basis of Suman and Bacon32. The peak in230Thxs0during the YD indicates a large particle influx and focusing at the coring site. The YD interval is also highlighted by a subsequent drastic change in the234U/238U activity ratio linked to distinct sediment sources; this unit is also characterized by its relatively high dolomite content in the silt and sand fractions, pointing to an Arctic-Canadian source for the detrital supplies. Figure 3: Geochemical and sedimentological data for core HLY0503-18MC. 230 Th xs0 , 230 Th/ 232 Th and 234 U/ 238 U are respectively represented in pink, purple and orange. The mean grain size is represented in dark green, the organic carbon content in light green, dolomite and calcite are respectively in light and dark blue for all size fractions. The initial excess of 230 Th ( 230 Th xs0 ) illustrated on top, represents the 230 Th produced through dissolved- 234 U decay in the water column and scavenged by sinking particles. It is calculated as the 230 Th in excess over the fraction supported by 234 U, in the sediment, with correction for radioactive decay since deposition. The horizontal dashed-line illustrating the 230 Th-production in the overlying water column is calculated on the basis of Suman and Bacon [32] . The peak in 230 Th xs0 during the YD indicates a large particle influx and focusing at the coring site. The YD interval is also highlighted by a subsequent drastic change in the 234 U/ 238 U activity ratio linked to distinct sediment sources; this unit is also characterized by its relatively high dolomite content in the silt and sand fractions, pointing to an Arctic-Canadian source for the detrital supplies. Full size image The above sedimentary features suggest a pulse in ice-rafted debris, at the study site, linked to enhanced sea-ice production and drifting from the Canadian Arctic area. A major drainage event from the LIS margin, the most plausible candidate indeed being here Lake Agassiz [17] , is seen as the trigger of this pulse in sea-ice production and export. Any northern drainage of Lake Agassiz, during this interval, had to occur in the corridor between the Cordilleran Ice Sheet and the LIS. Off the drainage outlet, such a meltwater pulse would have enhanced the production of sea ice 'labelled' by detrital particles carrying a mineralogical signature (dolomite) from the area. Sea-ice export through the central Arctic, through the Beaufort Gyre and then the Transpolar Drift, carried this signature as far as the Lomonosov Ridge, and had to result in an increase rate of sea-ice export through Fram Strait into the Greenland–Iceland–Norwegian seas and the North Atlantic. Also noteworthy is the fact that the end of YD interval (22 cm downcore MC-18) is marked by a major change in 234 U/ 238 U activity ratios ( Fig. 3 ). Above, 234 U is in deficit versus its parent 238 U, as is often observed in oxidized sub-surface sedimentary layers [26] , whereas below, near-equilibrium conditions prevail between the two isotopes. This suggests a change in sediment source and/or accumulation rate [27] . Because the 234 U-excess persists deeper in the core through the layer assigned to MIS 3, without being affected by their drastic difference in sedimentation rates, a change in sediment source seems more likely, following the YD. Here the possibility of a diagenetic uptake of uranium from sea water related to lower redox conditions is rejected since the organic carbon content is practically unchanged on both sides of this transition [28] . The change in sedimentary sources at the end of the YD interval suggests changes in the area of sea-ice production transporting sediment to the Lomonosov Ridge. During MIS 3 and the YD, the geochemical signature (presence of dolomite and high 234 U/ 238 U ratio) of Canadian margin material suggests a prominent influence of sea-ice from the Canadian Arctic with an active Beaufort Gyre ( Fig. 1 ). The absence of dolomite in the different size fractions during the Holocene, then suggests a significant reduction of Canadian sources and a dominant influence of material from Russian sources through direct Transpolar Drift supplies (see also ref. 20 ). On the basis of the Lomonosov ridge record, a drainage event with an Arctic-Canadian signature, at the onset of the YD is proposed. Earlier, Peltier et al . [29] and Peltier [6] , demonstrated that such a northern route for a freshwater pulse (through sea-ice export), likely linked to Lake Agassiz drainage accompanying some collapse of the Keewatin Dome of the LIS, would have been as efficient in 'shutting down' the AMOC. The hiatus matching MIS 2 (the last glacial maximum sensu lato ), suggests a complete interruption of sedimentation in the area, thus a sluggish Transpolar Drift (if any), with a thick pack ice occupying the central Arctic. The resumption of the sea-ice transport in the Central Arctic, due to the drainage event would have been responsible for enhanced sea-ice export through Fram Strait into the Nordic Seas, resulting in a slow-down of the AMOC. However, we must admit that inherent uncertainties of the marine 14 C chronology at the Allerød-YD transition added to poorly constrained 14 C-reservoir ages of Arctic waters, makes impossible to unequivocally identify the trigger mechanism responsible of the YD from such records. Study sites Core HLY0503-18 TC (88°27′ N; 146°34′ E; 2,598 m water depth, 117.8 cm in length) and core HLY0503-18 MC (88°26′ N; 146°41′ E; 2,654 m water depth, 47 cm in length) were retrieved in Lomonosov intrabasin during the HOTRAX 2005 expedition. Age model The age model used in this study is the age model published in Hanslik et al . [20] transposed from TC-18 to MC-18 based on 210 Pb profiles. Hanslik et al . [18] obtained eleven accelerator mass spectrometry 14 C ages on tests of planktic foraminifer assemblages ( Neogloboquadrina pachyderma ). These 14 C ages were calibrated using the Marine04 data set in OxCal 4.0 (with a 95% confidence interval). A Δ R =300 was applied on 14 C age from 0 to 16 cm, whereas Δ R =1,000 was applied deeper based on foraminifera abundances, as discussed in Hanslik et al . [20] Errors are 2 s.d. Two 14 C ages, deeper in the core, yielded ages beyond the OxCal calibration range. The Fairbanks0107 calibration curve was then used and the error corresponds to 1 s.d. (see Hanslik et al . [20] for details). U-series isotopes analysis Lead-210 isotopes were measured by alpha counting; uranium and thorium isotopes by multi-collector-inductively coupled plasma-mass spectrometry on bulk sediment. Initial 230 Th-excess values ( 230 Th xs0 ) in the deglacial to Holocene sections were simply calculated by subtracting 234 U-activities, and correcting for decay based on interpolated ages from calibrated ages. Sediment properties analysis Particle-size fractions were determined using a laser-diffraction particle-size analyser (LS13320 Beckman-Coulter) on bulk sediment, and grain-size statistics were processed with the Gradistat program. The silt fraction corresponds to the size fraction between 2 and 63 μm. Mineralogical assemblages were determined by X-ray diffraction using a Siemens D5000 with CoKα1,2 radiation and a Si detector. Semi-quantitative estimations (±1 σ ~5%) of the main mineral species were based on the area of the diffraction peak for each mineral corrected for quartz. The calcite and dolomite contents were measured in several fractions, including the >63 μm fraction, characteristic of ice-rafted sediment in deep-water marine environments. The organic carbon (Corg) content was determined by the acidification of total sediment with HCl 1N and elemental-C analysis of the residual fraction with a Carlo Erba elemental analyzer. Further details about methods can be found in Not and Hillaire-Marcel [22] . How to cite this article: Not, C. & Hillaire-Marcel, C. Enhanced sea-ice export from the Arctic during the Younger Dryas. Nat. Commun. 3:647 doi: 10.1038/ncomms1658 (2012).